Annotation of microsporidian genomes using transcriptional signals High-quality annotation of microsporidian genomes is essential for understanding the biological processes that govern the development of these parasites. Here we present an improved structural annotation method using transcriptional DNA signals. We apply this method to re-annotate four previously annotated genomes, which allow us to detect annotation errors and identify a significant number of unpredicted genes. We then annotate the newly sequenced genome of Anncaliia algerae . A comparative genomic analysis of A. algerae permits the identification of not only microsporidian core genes, but also potentially highly expressed genes encoding membrane-associated proteins, which represent good candidates involved in the spore architecture, the invasion process and the microsporidian–host relationships. Furthermore, we find that the ten-fold variation in microsporidian genome sizes is not due to gene number, size or complexity, but instead stems from the presence of transposable elements. Such elements, along with kinase regulatory pathways and specific transporters, appear to be key factors in microsporidian adaptive processes. Microsporidia are obligate intracellular parasites related to unicellular fungi. These microorganisms are ubiquitous in the animal kingdom, with more than 1,200 species invading a wide range of invertebrates and vertebrates [1] . Among these species is A. algerae , which was originally isolated from the larvae of the Anopheles stephensis mosquito [2] and has one of the broadest known host ranges [3] . This species infects both immuno-competent and immuno-compromised patients [3] , [4] . Furthermore, the mosquitoes co-infected with A. algerae and Plasmodium falciparum exhibit reduced Plasmodium development, suggesting that A. algerae enforces a biological defence against the causative agent of malaria [5] . Because of its impressive adaptive capacities (host spectrum, types of targeted cells and development over a large range of temperatures [6] ), A. algerae is an interesting model for understanding microsporidia adaptation and host interaction. In the microsporidia family, A. algerae has one of the largest genome sizes, estimated at 23 Mbp [7] (Megabase pairs), largely sufficient to potentially support the biological functions required to infect a large host spectrum. Its genome, however, is still poorly documented [8] . Moreover, comparative genomic analysis using currently available microsporidian genomic data from other fully sequenced genomes (that is, Encephalitozoon cuniculi [9] , Encephalitozoon intestinalis [10] , Enterocytozoon bieneusi [11] , [12] , Nosema ceranae [13] Octosporea bayeri [14] and more recently, Encephalitozoon romaleae [15] , Encephalitozoon hellem [15] , Nematocida parisii [16] and Nematocida sp1 [16] ) will provide a better understanding of specific host–parasite interactions and adaptation capacities. In genome annotation, gene structure prediction is one of the most important and exciting problems in computational biology [17] . Gene prediction methods based on extrinsic data, such as specially available orthologous gene sequences, have improved the specificity and complementary sensitivity of de novo prediction [18] . Such data, however, are not available for all genes; therefore, intrinsic approaches using ab initio gene prediction algorithms are required. These algorithms are based only on DNA sequence information [19] and display high sensitivity but low specificity. In general, ab initio methods do not ensure small open reading frame identification, and their sensitivity is reduced for rapidly evolving sequences [18] , as shown for microsporidian gene sequences [20] . Despite substantial progress in the past decade, current gene identification methods are not able to produce an in extenso catalogue of protein-coding genes [17] , [21] , [22] , [23] . In addition to gene prediction difficulties, the identification of translation initiation sites (TISs) also represents a major challenge. Our recent studies show that CCC-like or GGG-like motifs are present immediately upstream from the start codon [24] , [25] for all E. cuniculi genes as well as for genes encoding ribosomal proteins in the microsporidian species Antonospora locustae , E. bieneusi , A. algerae and N. ceranae [24] , [25] . The presence of these motifs in close proximity to the TISs was considered to significantly improve microsporidian genome annotation and re-annotation. Here we used this strategy to re-annotate the genomes of microsporidia E. intestinalis , E. cuniculi , N. ceranae and E. bieneusi , followed by the de novo annotation of the newly sequenced A. algerae genome. Finally, a high-quality comparative genomic analysis was conducted using newly predicted and re-annotated genes. 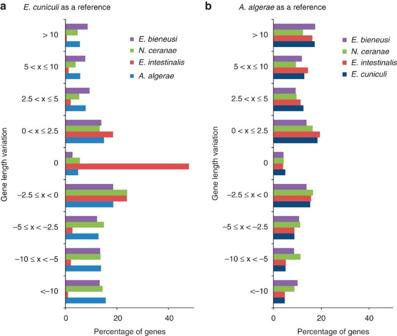Figure 1: Conservation of CDS length for the five microsporidian genomes. The CDS lengths of the orthologous genes were compared. Percentages of the difference (positive if the CDS is larger than its ortholog in the reference genome, 0 if lengths are equal and negative otherwise) were partitioned in nine different classes. (a)E. cuniculias the reference for CDS length. (b)A. algeraeas the reference for CDS length. Re-annotation of four published genomes Taking advantage of CCC-like or GGG-like motifs, the positions of the E. intestinalis TISs were revised for 148 predicted coding DNA sequences (CDSs) ( Table 1 ; Supplementary Data 1 ) and validated by using the Kozak sequence bias. After the re-annotation, we observed 42.56% of A and 42.56% of G in the +4 position from the TIS position and 50% of A in the +5 position, compared with 29.05% of A and 24.32% of G in the +4 position and 28.37% of A in the +5 position for most likely falsely predicted TISs. These values were in accordance with the Kozak sequence bias of E. cuniculi [24] and reinforced the pertinence of the E. intestinalis TIS revision. Moreover, new spliceosomal introns were characterized in nine CDS ( Supplementary Data 1 ). With this method, several sequence frameshifts and sequencing errors responsible for the false predictions in six genes were also identified. In addition, the TIS re-annotation strategy revealed that two predicted genes were erroneous in the reading frame, leading to a total of eight badly predicted genes ( Supplementary Data 2 ). Table 1 Re-annotation of four microsporidian genomes. Full size table Surprisingly, for four protein-coding genes (UniProtKB accession codes Eint_050670, Eint_071680, Eint_081300 and Eint_101000) with orthologous sequences in another microsporidian, no conventional CCC-like or GGG-like signals were present in the TIS upstream region (50 bases), but a strong adenine/thymine-rich sequence (between 74 and 78%) was present. 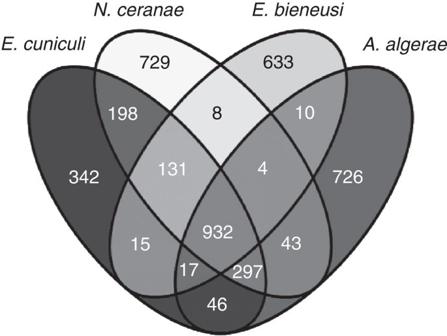Figure 2: Protein-coding gene distribution among the four microsporidian species. Venn diagram showing the distribution of shared genes amongE. cuniculi,N. ceranae, E. bieneusiandA. algerae. For the N. ceranae and E. bieneusi genomes comprising a high AT content (74% and 76%, respectively, Table 2 ), a significant number of TISs, validated by comparative analysis, was also not preceded by a CCC-like or GGG-like motif but instead by an AT rich region (approximately 90%). The sequence signals allowed us to revise 309 and 245 AUG initiation codons of the predicted CDSs from the N. ceranae and E. bieneusi genomes, respectively ( Table 1 and Supplementary Data 1 ). In contrast to the E. intestinalis and E. cuniculi species, however, our prediction for these species could not be validated by the Kozak sequence bias. In the N. ceranae genome, two new spliceosomal introns were found; in the N. ceranae and E. bieneusi genome sequences, 29 and 15 unidentified frameshifts and two and four unidentified sequence errors, respectively, were also identified ( Supplementary Data 1 ). Table 2 General characteristics of Anncaliia algerae and other microsporidian genomes. Full size table This TIS re-annotation based on specific signals allowed the characterization of 76 and 168 wrongly predicted genes ( Supplementary Data 2 ). The E. bieneusi genome also presented 387 genes corresponding to 253 contigs that do not harbour the conventional signals upstream from the TIS but encode proteins with orthologous sequences in the non-redundant NCBI protein database ( Supplementary Data 3 ). The BLASTP results revealed that the best hits are generally obtained with bacterial sequences belonging to the Pseudomonas genus. Finally, the N. ceranae sequence similarity search and clustering approaches identified 475 genes that encode proteins corresponding to transposable elements (TEs, Supplementary Data 4 ). The genomic comparative analysis and TIS re-annotation of the CDSs from E. intestinalis, N. ceranae and E. bieneusi allowed the revision of 97 AUG initiation codons for the E. cuniculi genome, compared with the previous re-annotation [24] . The re-annotations also confirmed the presence of three additional spliceosomal introns characterized and validated by a rapid amplification of cDNA ends-PCR (RACE–PCR) approach [26] ( Supplementary Data 1 ). In conclusion, the identification of these particular microsporidian upstream CDSs signals ensures an accurate revision of already-predicted genes. To identify the unpredicted genes from the four annotated microsporidian genomes, we initially used the extrinsic approach using predicted orthologous genes, resulting in 33, 14, 94 and 46 new genes identified in the E. cuniculi, E. intestinalis , N. ceranae and E. bieneusi genomes, respectively ( Supplementary Data 5 ). As extrinsic data were not available for all the genes, the intrinsic approach based on the identification of the TIS in an appropriate context, the GC content of the CDS and the presence of a poly-adenylation signal close to the stop codon was applied. We also identified 77 additional genes in the E. cuniculi genome, among which 70 possessed orthologs in the E. intestinalis genome that had not been previously detected. [10] Thirty-one also presented unpredicted orthologs in the N. ceranae and/or E. bieneusi genomes, suggesting that these are real and conserved genes. Finally, we found 12 encoded proteins with motifs described in the Interpro database ( Supplementary Data 5 ). To validate our results, the Kozak sequence bias was assessed for the 110 (33+77) newly identified E. cuniculi genes. Analysis shows 33.33% of A and 45.95% of G in the +4 position as well as 45.95% of A in the +5 position, which reinforces the pertinence of our prediction. Application of the same intrinsic strategy for the E. intestinalis genome annotation allowed us to describe 70 additional genes, leading to a total of 84 unpredicted genes in this genome ( Table 1 ; Supplementary Data 5 ). All of these genes present the conventional CCC-like or GGG-like signals upstream from the TIS and the same bias in their Kozak sequences (+4: 35.71% A and 45.24% G, +5: 52.38% A). Finally, in N. ceranae and E. bieneusi , 198 and 24 new genes were characterized, leading to a total of 292 and 70 unpredicted genes, respectively ( Table 1 ). For the intrinsic predicted genes in N. ceranae and E. bieneusi , 29 and 14, respectively, harbour an unpredicted orthologous gene in another microsporidian species, and for 27 and 11, respectively, an Interpro domain was detected ( Supplementary Data 5 ). None of the 70 newly predicted genes identified in E. bieneusi corresponded to core carbon metabolism, thereby confirming that this species has no fully functional pathway to generate ATP from glucose [12] . To reinforce our bio-informatic re-annotation, we conducted 5′RACE–PCR experiments on several E. cuniculi genes that had previously been incorrectly predicted, not predicted or had been with falsely predicted TISs. As 5′ untranslated regions may be highly reduced by identifying transcriptional start sites, the TISs located in close proximity to the transcriptional start site could be characterized. For the 17 newly predicted genes studied, the 5′RACE–PCR fragment sizes were in accordance with the predicted TISs of these genes ( Supplementary Fig. S1 , gels 1–2). These fragments allowed the validation of the newly proposed TIS for the five genes studied ( Supplementary Fig. S1 , gel 3). Finally, the absence of DNA fragments of the expected size confirmed that the 11 previously predicted genes do not exist ( Supplementary Fig. S1 , gel 4). Draft of A. algerae genome Approximately 110 Mb of DNA sequence was obtained from random shotgun sequencing using the Sanger method, resulting in an estimated 4.77 coverage of the A. algerae genome, which is estimated at 23 Mbp [7] . The reads were assembled into 8,427 contigs ( Supplementary Data 6 ) with a N 50 length of 2.209 kb. The genomic G+C content (24%) was significantly lower than that observed in E. cuniculi or E. intestinalis but similar to that of N. ceranae or E. bieneusi ( Table 2 ). The coding capacity and structure of the A. algerae genome were determined using both extrinsic and intrinsic approaches, and 6,058 partial or complete CDSs were subsequently identified. Owing to the high sequence variability, particularly in the intergenic regions (single nucleotide (nt) and insertion/deletion) excluding sequencing errors due to Sanger sequencing, we were unable to assemble different contigs containing genes encoding similar proteins, as illustrated in Supplementary Fig. S2 . Genes encoding proteins harbouring >97% of identity were clustered, allowing the identification of 2,075 gene clusters. Each encoding protein may possess the same biological function ( Supplementary Data 7 ). Of these 2,075 genes, 698 (33.64%) were located on contigs including a TE, a sequence element commonly found in microsporidia with large genomes [8] , [13] , [14] , [27] , [28] , [29] , [30] , [31] and already described for this species [8] . Furthermore, in rare cases, contigs including similar genes harboured different genomic organizations, but, in all cases, the changes were due to the integration of transposable elements. In addition, 13.4% of all genes showed synteny with those of E. cuniculi ( Supplementary Data 8 ). The seven short introns observed in the A. algerae genome ( Table 2 ) were all located in protein ribosomal genes ( L44, S30, L37a, S12, S26, S3A and L1 ). Four of them were present as an orthologous gene with an intron in E. cuniculi and/or in E. intestinalis , but none were present in N. ceranae or E. bieneusi. Concerning protein sizes, TIS re-annotation allowed for an accurate comparison of the E. cuniculi , E. intestinalis , N. ceranae , E. bieneusi and A. algerae proteomes. The analysis showed that 60.9% of A. algerae proteins were smaller than their orthologs in E. cuniculi and E. intestinalis ( Fig. 1 ). When compared with the proteins of N. ceranae and E. bieneusi , 47.8 and 52.4% of the proteins of A. algerae were larger, whereas 47.8 and 43.3% were smaller. Figure 1: Conservation of CDS length for the five microsporidian genomes. The CDS lengths of the orthologous genes were compared. Percentages of the difference (positive if the CDS is larger than its ortholog in the reference genome, 0 if lengths are equal and negative otherwise) were partitioned in nine different classes. ( a ) E. cuniculi as the reference for CDS length. ( b ) A. algerae as the reference for CDS length. Full size image Comparative genomic analysis The comparative genomic analysis was conducted on the E. cuniculi , N. ceranae , E. bieneusi and A. algerae proteomes. Because the E. intestinalis proteome ( Supplementary Data 9 and 10 ) was very similar to that of E. cuniculi , with only 28 additional proteins detected [10] , it was not included in the following analysis for simplicity and to improve the readability of our presentation. For these 4 microsporidian proteomes, 1,978 ( Supplementary Data 11 and 12 ), 2,342 ( Supplementary Data 13 and 14 ), 1,750 ( Supplementary Data 15 and 16 ) and 2,075 ( Supplementary Data 17 and 18 ) non-redundant proteins were found ( Table 2 ), with a core proteome composed of 932 proteins ( Fig. 2 ; Supplementary Data 19 ). In this core proteome, 141 proteins were putatively specific to the entire microsporidian phylum because they were absent in any other eukaryotic phylum ( Supplementary Data 20 ). Motif Alignment and Search Tool (MAST) and Multiple Em for Motif Elicitation (MEME) analyses [32] showed that 41 proteins were encoded by genes that harbour an AAATTT-like motif or AT-rich sequence upstream of their TISs, both sequences believed to be regulatory elements involved in gene expression enhancement [24] , [33] . Among these 41 genes, we found proteins contributing to specific major structural and/or physiological characteristics of the parasitic cell, such as the spore wall, polar tube formation and the parasite-host surface interactions. Therefore, we focused our attention on the structural proteins to identify potential addressing signals or transmembrane domains. These analyses not only allowed for the identification of already described polar tube and spore wall proteins but also of seven additional proteins predicted to be exported and/or with trans-membrane helices ( Supplementary Data 21 ). Figure 2: Protein-coding gene distribution among the four microsporidian species. Venn diagram showing the distribution of shared genes among E. cuniculi , N. ceranae, E. bieneusi and A. algerae . Full size image The functional annotation executed for each microsporidian species showed striking similarities between the microsporidian species in the gene ontology categories ( Fig. 3 ). The A. algerae proteome, however, displayed a significant overrepresentation of protein phosphorylation and trans-membrane transporters ( Fig. 3 ). In eukaryotes, phosphorylation is a post-translational modification involving kinases. Phosphorylation has a crucial role in most cellular processes, such as cell cycle, cell growth, receptor activations, metabolic pathways, enzyme activities, protein activation/inhibition and cytoskeletal organization. 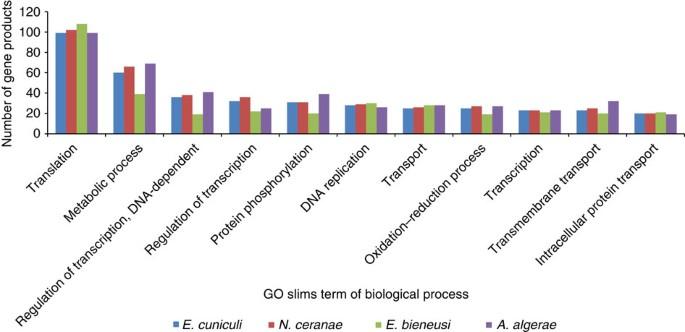Figure 3: Distribution of microsporidian proteins among biological processes. Only major biological process ontology categories forE. cuniculi,E. bieneusi,N. ceranaeandA. algeraeare given. These data reflect absolute gene numbers in each major category. The ordinate represents the number of CDSs assigned to the corresponding category. Comparison of the kinomes revealed that most kinases found in E. cuniculi were present in all microsporidia but that the A. algerae kinome presented a higher diversity ( Table 3 ). The large number of proteins belonging to the CMGC family were the most important ( Table 3 ). Although some kinases involved in cell cycle control are absent in the A. algerae proteome, their presence in other microsporidians suggest that they form part of the genomic fractions that are lacking in A. algerae . Fourteen kinases absent in E. cuniculi are found in N. ceranae and A. locustae , both microsporidia that infect insects. These data indicate that they could be involved in the regulation of the insect–parasite cycle or infection. Seven A. algerae -specific kinases with homology to yeast kinases were also found. Finally, one GCN2 (general control non-de-repressible 2)-like kinase, as well as two mitogen-activated protein kinase kinase kinase (MAPKKK) proteins belonging to the STE family (Ste11 and Ste20), were identified only in the A. algerae proteome ( Table 3 ), suggesting that these kinases could be related to A. algerae physiology or life cycle. To check that they were not contaminants, both sequences were amplified by PCR ( Supplementary Fig. S3 ). Figure 3: Distribution of microsporidian proteins among biological processes. Only major biological process ontology categories for E. cuniculi , E. bieneusi , N. ceranae and A. algerae are given. These data reflect absolute gene numbers in each major category. The ordinate represents the number of CDSs assigned to the corresponding category. Full size image Table 3 Comparative microsporidian kinome analysis. Full size table Another overrepresented GO category in the A. algerae proteome is the transporters. To improve our knowledge about host interaction/dependency, microsporidian transporter repertoires were compared ( Fig. 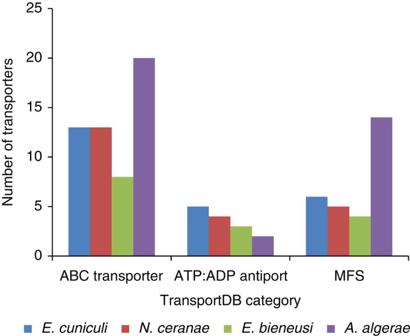Figure 4: Comparison of microsporidian transporter proteins. Transport proteins belong to the ATP-binding cassette (ABC) family, the ADP:ATP antiport family and the major facilitator superfamily (MFS). They have been identified using TransportDB. The ordinate represents the number of CDSs assigned to the corresponding category. 4 , Table 4 ). As with all microsporidia, A. algerae features several transporters that are involved in nutrient salvage from the host. Twenty ATP-binding cassette family transporters, two ADP/ATP transporters and 15 sugar or nt-sugar transporters belonging to the major facilitator super-family were characterized ( Fig. 4 , Table 4 ). Figure 4: Comparison of microsporidian transporter proteins. Transport proteins belong to the ATP-binding cassette (ABC) family, the ADP:ATP antiport family and the major facilitator superfamily (MFS). They have been identified using TransportDB. The ordinate represents the number of CDSs assigned to the corresponding category. Full size image Table 4 Comparative microsporidian transportome analysis. Full size table A re-annotation was undertaken for four microsporidian species by coupling the specific signals located upstream of TIS identification to conventional gene prediction methods. Our results highlighted the fact that conventional approaches used to annotate these genomes are not sufficient. The assumption made by many gene predictors, wherein they consider the first AUG present in an open reading frame as the TIS, is not always valid. The present work demonstrates that CCC-like or GGG-like sequence motifs and also AT-rich regions upstream in some N. ceranae and E. bieneusi genes, allow the unambiguous positioning of the TIS. Several arguments support the presence of badly predicted genes: (i) they do not possess a TIS with the relevant upstream signals, and in some cases, no AUG codons were identified; (ii) some overlap fully or partially with other predicted genes, and in other cases the genes have not been assigned to the right strand; (iii) poly-adenylation signals near the termination codon necessary to ensure mRNA 3′-end processing are absent [24] ; and (iv) comparative genomic analyses with the non-redundant protein database of NCBI do not allow the identification of similar sequences. In addition, some E. bieneusi erroneous CDSs were also predicted in low complexity DNA sequences or initiated under a leucine codon, reflecting the drawback of using the GLIMMER prokaryotic version [11] . Despite the authors' efforts, some bacterial sequences were still present because of the insufficiently stringent criteria used to eliminate them [11] . The similarity and clustering approaches identified the putative TE sequences, which had previously been predicted to exist in the N. ceranae genome. Moreover, five multi-gene families, each with at least ten members, have been described and considered to be uncharacterized TEs [15] . To confirm the fact that these genes correspond to TEs, we have shown that some members of these five families harbour degenerate sequences corresponding to relic elements similar to the majority of the TE-derived sequences described [34] . For this reason, members of these multi-gene families can be included in the putative TE sequences. Our dedicated intrinsic and extrinsic approaches have also identified additional genes in the four microsporidian species. The high proportion of previously unpredicted genes for N. ceranae and E. bieneusi can be explained by the annotation strategies. Genes with known homologues were identified with the BLASTX programme using an expect value cutoff of 1e −15 and 1e −5 (refs 11 , 13 ). The two expect values used, however, are too low to ensure the detection of short sequences and/or highly divergent orthologs due to the high rate of protein-sequence evolution in the microsporidian phylum [20] . For the E. intestinalis genome annotation [10] , the authors used BLAST approaches with parameters more suitable to the effective identification of orthologs, and they detected 16 new genes previously unannotated in the E. cuniculi genome. These innovative, efficient and reliable annotation strategies were then used to enable the annotation of the A. algerae genome. We identified 6,058 complete or partial CDSs, some of which encode proteins harbouring >97% of identity and, in more than half the cases, identify more than two different gene sequences. Furthermore, higher sequence variability (insertion/deletion events) has been observed in intergenic regions of genes encoding similar proteins. Such sequence variability has also been previously observed by sequencing cloned PCR products from A. algerae and also A. locustae [35] . Sequence polymorphisms have recently been described in the Nematocida genus [16] . Indeed, these authors have identified SNPs preferentially located in coding regions that generate synonymous codons. Because the reference and alternate allele are each supported in roughly equal proportions, these Nematocida species appear to be diploid and heterozygous. For A. algerae , because more than two similar sequences have been identified for numerous genes, three hypotheses have been proposed to explain such a situation. All of the evidence points to significant regions of the genome, if not the entire genome, either being duplicated or existing in two copies as part of the diplokaryotic nature of the organism. These results may indeed be due to the polyploidy of the A. algerae genome and/or to the duplication of large DNA sequences, including several genes. Furthermore, the hypothesis that this sequence variability arises from the presence of heterogeneous populations in the cultures cannot be completely excluded. It is likely that future (third or subsequent) sequencing generations will sequence long fragments (several tens of kb) on single molecule extracts from a unique cell or clonal population; this method will be helpful in making conclusions concerning such complex genome situations. Gene-order conservation between A. algerae and E. cuniculi is close to that observed between A. locustae and E. cuniculi (13%), despite the fact that these microsporidia are distantly related [35] . In microsporidian genomes, this unexpected degree of synteny is in agreement with a low rate of genomic reorganization, most likely due to a low rate of recombination. Nevertheless, an exploration of genomic data shows that a significant proportion of A. algerae genes are in close proximity to the TEs and that the genomic organization is quite different from that found in the E. cuniculi , E. intestinalis , N. ceranae and E. bieneusi genomes ( Table 2 ). For N. ceranae and E. bieneusi , even though the TEs and repeat sequences have been identified, the genes are generally closely clustered in large DNA regions. The genomic organization of A. algerae is not unique to microsporidia and is similar for O. bayeri , a species with a genome size estimated at 24 Mbp and for which the high sequencing coverage (34.2–37.2x) allows assembly of reads into 41,804 contigs with an average length of only 320 bp [14] . In conclusion, in large microsporidian genomes, genes scattered across the entire genome could be separated by TEs or by repeat regions, leading to highly variable gene densities across the genome. Furthermore, we have identified contigs within similar genes that show different genomic organization; such changes are due to the integration of a transposable element. The present analyses suggest that microsporidian species may have been derived from an ancestor organism with high gene compaction and that due to the acquisition of DNA (that is, TEs), some have evolved towards larger genomes. Furthermore, such genome invasion by TEs has recently been described for Blumeria graminis , a filamentous plant pathogenic fungus [36] . In this species, the TEs were evenly distributed throughout the genome, and the protein-coding genes are, consequently, in small clusters, as in the A. algerae genome. Such organisms, therefore, possess a higher genome plasticity to ensure adaptation to the various environments in which they develop [37] . This adaptation is also the case for A. algerae , which presents a large host spectrum. The present analyses suggest that the number of introns is not responsible for genome compaction because no intron could be identified in the E. bieneusi genome and because only a small number was observed for the other microsporidian species, independent of whether they had a large genome. Moreover, all of the additional introns in E. cuniculi [26] characterized by RACE–PCR were also identified by their homologs in E. intestinalis , whereas they were absent in those of the species N. ceranae , E. bieneusi and A. algerae that had larger genomes. Finally, the present analyses show that genome size variation in microsporidia is not correlated with the protein-encoding gene size. A. algerae genes are generally shorter than those found in E. cuniculi and E. intestinalis , whereas genes in O. bayeri , characterized by a genome of 24 Mbp proteins, are on average larger than the orthologs in E. bieneusi and E. cuniculi [14] . N. ceranae harbours the most important number of single copy protein-coding genes identified. However, only 38 tRNA genes were identified in A. algerae , whereas 44 have been identified in the other microsporidian species studied ( Table 2 ). In addition, an evaluation of the gene distribution shows the absence of 131 protein-coding genes in A. algerae compared with that of E. cuniculi , N. ceranae and E. bieneusi ( Fig. 2 ); this absence suggests that sequencing coverage was insufficient for the complete genome. The lack of 297 protein-coding genes in the E. bieneusi genome might convey a similar conclusion. Nevertheless, the analyses suggest that the gene number for these two species may be close to that of N. ceranae . Large microsporidian genomes, therefore, do not necessarily encode significantly more genes than do smaller ones, and the complexity of the proteome is not a major factor contributing to genome size variation. Most of this variation can be attributed to length variations of intergenic regions and to the number of repeat sequences and TEs. In addition, genome size variations in microsporidia may also be a consequence of variations in the size of telomere repeats, as suggested by the O. bayeri sequencing project [16] . Comparative genomic analyses allowed the identification of a core proteome composed of 932 proteins. This core genome may be more important mainly because the sequencing coverage was insufficient to obtain the complete genome of A. algerae and E. bieneusi . It is likely, therefore, that a large part of the 131 and 297 genes not identified only in the A. algerae and E. bieneusi genomes should be included in this microsporidian core genome. Furthermore, in some cases, it is not possible to identify orthologous sequences using only similarity criteria due to the evolution rate of microsporidian sequences. For example, some polar tube-encoding genes were characterized only by taking into account the synteny [38] . Comparative genomic analyses were then based on highly expressed microsporidian-specific genes encoding membrane-associated proteins (cell surface proteins, exported proteins, polar tube proteins, proteins exposed to the host immune system and transporters). All of these proteins were good candidates for experimental investigation to decipher their roles, particularly those proteins involved with spore architecture, and to better understand the invasion process and/or the relationship of these microsporidia to their hosts. Finally, studies were focused on functionally annotated genes and, more particularly, on those overrepresented in the A. algerae genome. The A. algerae kinome presents some specific characteristics that can be related to its physiology or its life cycle. For example, a GCN2-like kinase has been identified that is also present in A. locustae , another insect microsporidia. GCN2p is involved in eiF2α phosphorylation, leading to translation inhibition in nutrient starvation conditions in yeast [39] as well as in other intracellular eukaryotic parasites [40] , [41] , [42] . Furthermore, Ste20 and Ste11 belonging to the MAPKKK pathway were also identified. Both proteins are known to have various functions in signalling pathways, morphogenesis, pathogenesis, filamentous growth under poor nutritional conditions and in response to high osmolarity adaptation [43] , [44] . The data indicate that, as in yeast, A. algerae presents kinases involved in stress response. Through these responses, the parasite adapts to distinct physiological environments found in their insect and mammalian hosts, such as stress situations. In the A. algerae kinome, the rest of the components of the MAPK regulatory pathway, such as Ste7 and the kinase phosphorylated by Ste11, are absent and can be explained also by sequences being too divergent to be identified or because the genome was not fully sequenced. A. algerae presents the large transporter repertoire necessary to acquire amino acids and nutrients from the hosts. Such diversity could be related to the fact that A. algerae is able to infect both mammals and insect hosts. This diversity also suggests an increased host dependency, which is not in accordance with O. bayeri proteomic data, and suggests an increased genome complexity related to reduced host dependency [16] . Furthermore, the metabolic patterns of how the insect and mammalian stages of the parasite acquire amino acids and other nutrients are unknown, suggesting that the detected transporter genes need to be elucidated by further bench work on the precise metabolic pathways. Finally, A. algerae presents one of the largest repertoires of kinases and transporters; this large repertoire is most likely related to the broad host range known to be infected by this microsporidia. As these parasites rely on scavenging from the host via a series of transporters, the transporter repertoire could also be exploited for antimicrosporidia chemotherapy. DNA production and sequencing The A. algerae isolate used in this study was kindly provided by Pr W. A. Maier (University of Sigmund-Freud, Bonn) and corresponds to the microsporidium isolated by Dr A. Undeen from its original mosquito host ( A. stephensi ). Spores were collected weekly from infected HFF cell cultures, and DNA was extracted according to Belkorchia et al . [9] A whole genome sequencing strategy and a hierarchical shotgun sequencing strategy were then applied. DNA was fragmented by mechanical shearing or by Sau 3A partial digestion and cloned into pcdna2.1 (Invitrogen), pCNS (pSU18 derived) and pBeloBAC11 vectors. Recombinant plasmids and BAC DNAs were purified and end-sequenced using dye-terminator chemistry on Applied Biosystems 3730 automatic sequencers. Sequence preprocessing and assembling processes were realized using the Staden software package ( http://staden.sourceforge.net/ ). Owing to the sequence polymorphism, the assembly process was performed using stringent criteria. Sequence quality was evaluated using the Phred algorithm. Poor-quality sequences were deleted with the quality clip algorithm; Phred values with high thresholds were used to exclude all poor-quality sequences (the quality value was 28 averaged over 50 bases). The assembly was realized using the normal shotgun assembly algorithm of the gap4 software in four steps using the following thresholds: (1) minimum initial match of 300 nt and maximum percent mismatch of 0%; (2) minimum initial match of 200 nt and maximum percent mismatch of 0%; (3) minimum initial match of 100 nt and maximum percent mismatch of 0%; (4) minimum initial match of 100 nt and maximum percent mismatch of 1%. The A. algerae contig sequences are available from EMBL under accession codes CAIR01000001 to CAIR01008427. Re-annotation of four published genomes Genome sequences were extracted from the EMBL database (accession codes for E. cuniculi : AL391737, AL590442–AL590451; for E. intestinalis : CP001942–CP001952; for N. ceranae : ACOL01000001–ACOL01005465; and for E. bieneusi : ABGB01000001–ABGB01001743). Putative erroneous-predicted TISs from E. cuniculi and E. intestinalis were revised by searching for CCC-like or GGG-like motifs in the 30 nts upstream of the AUG initiation codons. Newly predicted TISs for these two species were validated by analysing the Kozak sequence bias. Nt frequencies at the +4 and +5 positions were compared between the newly predicted TISs and those computed in a previous study on E. cuniculi [24] . For the N. ceranae and E. bieneusi genomes without CCC-like or GGG-like motifs, compositional bias of the 30 nts upstream of the TISs was evaluated, and an AT content >80% was considered as an additional criterion to ensure the revision of start codons for these two species. A BLASTP [45] analysis of the N-terminal protein sequences was performed for each of the newly predicted TISs from the four microsporidian genomes to validate our results. A BLOSUM45 substitution matrix was chosen, and low-complexity filters were suppressed (-F F) to identify distant homologies. Identification of unpredicted genes from these previously annotated genomes was performed using both an extrinsic and an intrinsic approach. The extrinsic strategy relies on a TBLASTN analysis, comparing each previously annotated protein against other microsporidian sequences. BLAST parameters were tuned to identify distant homologues. The substitution matrix was set to BLOSUM45, and low-complexity filters were turned off. The intrinsic strategy consists of a systematic analysis of all intergenic sequences to detect putative CDSs and start codons with a CCC-like motif, a GGG-like motif or an AT content >80% in the 30 nts upstream. Validation for E. cuniculi and E. intestinalis was performed using Kozak's sequence bias. For each re-annotated microsporidian genome, two Supplementary Data were produced containing gene and protein sequences deduced from genes without sequencing errors (frameshift or stop codon introduction) as follows: E. intestinalis ( Supplementary Data 9 and 10 ); E. cuniculi ( Supplementary Data 11 and 12 ); N. ceranae ( Supplementary Data 13 and 14 ); and E. bieneusi ( Supplementary Data 15 and 16 ). Re-annotation validation by 5′RACE–PCR experiments Total RNA was extracted after 2 days from E. cuniculi -infected HFF and purified using the RNeasy Midi Kit (Qiagen) as previously described. The 5′RACE–PCR experi-ments were conducted to amplify the cDNA ends using the SMARTerTM RACE Amplification kit (CLONTECH) according to manufacturer's recommendations. The experiments were performed on the 11 genes considered as wrongly predicted as well as on several newly predicted genes (17) and on some with mispredicted TISs (5). For the newly predicted genes, we focused our attention on the genes that were also unpredicted in the other three re-annotated microsporidian genomes. We analysed five newly predicted genes in the four genomes, five genes absent only in the E. bieneusi genome, two genes absent only in the N. ceranae genome and five genes present only in E. cuniculi and E. intestinalis. The primers used and the 5′RACE–PCR results are presented in Supplementary Fig. S1 . Structural annotation of A. algerae To perform the structural annotation of A. algerae , a comparative analysis of the E. cuniculi , N. ceranae and E. bieneusi annotated microsporidian proteomes was conducted using the TBLASTN program. To identify the small proteins, a BLOSUM45 substitution matrix was chosen, and low-complexity filters were suppressed. TBLASTN analyses were manually validated to take into account genes with frameshifts due to sequencing errors. Orphan genes specific to A. algerae were found using an intrinsic approach based on the CCC-like and GGG-like motifs upstream of the TISs. Moreover, as A. algerae harbours an AT-rich genome, these data were considered to identify the unpredicted genes. Repetitive and transposable elements were removed using a BLASTX analysis. Each newly predicted CDS was compared against Repbase release 16.11 (ref. 46 ). The substitution matrix was set to BLOSUM45, and low-complexity filters were turned off. Distant homologs of these elements were identified using a single-linkage clustering approach. The clustering thresholds were chosen as follows: 50% identity (-S 50) between two amino acids sequences (-p T) and length coverage >50% (-L 0.5) for both sequences (-b T). Overrepresented gene families obtained after the BLASTCLUST clustering step were analysed, and the clusters containing TEs were removed. Finally, the tRNAs were predicted using the tRNAscan SE program [47] . Comparative genomic analysis and functional annotation An 'all-versus-all' BLASTP comparison of the predicted protein sequences within each of the four genomes was conducted. On the basis of the best BLASTP hits, orthologous relationships were established between the protein sequences of E. cuniculi , N. ceranae , E. bieneusi and A. algerae . To improve the accuracy of our orthologous prediction, especially for ambiguous results, local alignments obtained with BLASTP analyses were manually validated, and protein sizes and/or synteny were also checked. A Venn diagram was drawn using the Venny web service [48] . An intrinsic prediction of protein functions was performed using InterproScan 4.8 [49] . On the basis of the comparative analyses conducted in the structural annotation step, a functional annotation transfer was performed between orthologs. Protein sequences of genes with frameshift mutations were reconstructed. Gene ontologies and Interpro signatures were then automatically extracted. SignalP programme version 4 ( www.cbs.dtu.dk/services/SignalP/ ) [50] , the HMMTOP programme version 2.0 ( www.enzim.hu/hmmtop ) [51] , TMPRED ( http://www.ch.embnet.org/software/TMPRED_form.html ) and the PSORT II algorithm ( www.psort.nibb.ac.jp/form2.html ) [52] were used to predict the signal peptide, transmembrane helices and protein localization. For post-translational modifications, we looked for GPI anchors ( http://mendel.imp.ac.at/sat/gpi/gpi_server.html ) [53] , myristoylation ( http://web.expasy.org/myristoylator/ ) [54] , palmitoylation ( http://csspalm.biocuckoo.org/ ) [55] and prenylation ( http://mendel.imp.ac.at/sat/PrePS/index.html ) [56] . To model the kinases into families, Kinomer v.1.0 ( http://www.compbio.dundee.ac.uk/kinomer/bin/runHMMer.pl ) [57] was used. The transporter family comparisons were performed using the TransportDB database ( http://www.membranetransport.org/ ) [58] . MAPKKK amplification To check that the MAPKKKs were really A. algerae sequences, we amplified both genes, which are located on contig CAIR01007327 and CAIR01007503 by PCR using specific primers (sense primer 5′-AGGCACTAGGTAGAACATCAACAGG-3′; reverse primer 5′-GGGAATTCTCATCTTTAACCACTGGC-3′ for CAIR01007327; sense primer 5′-GAATTTATTGGAACAATTGTTAGAAGG-3′ and reverse primer 5′-GTTTTTCTGCTGTAGGTCTTTCG-3′ for CAIR01007503). Accession codes Contigs sequences have been submitted to EMBL database with accession codes CAIR01000001 – CAIR01008427 . All information is also available in the Supplementary Data. How to cite this article: Peyretaillade, E. et al . Annotation of microsporidian genomes using transcriptional signals. Nat. Commun. 3:1137 doi: 10.1038/ncomms2156 (2012).